Efficient and tuneable photoluminescent boehmite hybrid nanoplates lacking metal activator centres for single-phase white LEDs White light-emitting diodes (WLEDs) are candidates to revolutionize the lighting industry towards energy efficient and environmental friendly lighting and displays. The current challenges in WLEDs encompass high luminous efficiency, chromatic stability, high colour-rending index and price competitiveness. Recently, the development of efficient and low-cost downconverting photoluminescent phosphors for ultraviolet/blue to white light conversion was highly investigated. Here we report a simple route to design high-efficient WLEDs by combining a commercial ultraviolet LED chip (InGaAsN, 390 nm) and boehmite (γ-AlOOH) hybrid nanoplates. Unusually high quantum yields ( η yield =38–58%) result from a synergic energy transfer between the boehmite-related states and the triplet states of the benzoate ligands bound to the surface of the nanoplates. The nanoplates with η yield =38% are able to emit white light with Commission International de l’Eclairage coordinates, colour-rendering index and correlated colour temperature values of (0.32, 0.33), 85.5 and 6,111 K, respectively; overwhelming state-of-the-art single-phase ultraviolet-pumped WLEDs phosphors. The application of current mercury-based light sources for illumination will be limited due to the environmental concerns. Recently, solid-state phosphor white light-emitting diodes (WLEDs) have received considerable attention. WLED devices exhibit extra-long lifetime, excellent thermal resistance, higher luminous efficiency and lower power consumption compared to mercury-based fluorescent lamps [1] , [2] , [3] , [4] , [5] , [6] , [7] , [8] , [9] , [10] , [11] , [12] , [13] , [14] , [15] . There are at least three methods to generate white light in WLEDs: (i) the combination of three primary red, green and blue LEDs (RGB-WLED); (ii) the blue chip (450–470 nm)-pumped WLED (BLUE-WLED) and (iii) the near-ultraviolet chip (350–420 nm)-pumped WLED (ultraviolet WLED) [2] , [3] , [4] . The most efficient WLED is a combination of a blue LED chip and YAG:Ce 3+ yellow-emitting phosphor. The main disadvantages of such WLED are the poor colour-rendering index (CRI) and the low stability of correlated colour temperature (CCT) that varies with drive voltage and the phosphor coating thickness [16] . Ultraviolet-pumped WLEDs have huge potential because they are easy to manufacture, the white light emission is only due to the downconverting phosphors, they exhibit a low colour point variation as a function of the forward-bias currents and they have superior temperature stability [5] , [6] , [7] , [8] , [9] , [10] , [11] , [12] . Moreover, as the human eyes are insensitive to ultraviolet radiation, the white colour is independent of the pumping LED and thickness of the phosphor layer [15] . In ultraviolet-pumped WLEDs, multilayers of phosphors with distinct colour emission are generally used [14] , [15] , [16] , [17] , [18] , [19] . However, due to the reabsorption of light within the multicomponent phosphors, non-uniformity of luminescent properties with colour altering and a decrease of luminous efficiency are generally observed [2] , [20] . For these reasons, an ultraviolet-pumped WLED based on a single layer of a full-colour-emitting phosphor would be highly advantageous, promising very small colour variations, high CRI and low cost [5] , [6] , [8] , [9] , [10] , [11] , [12] , [13] , [18] , [21] , [22] . Nevertheless, actual downconverting phosphors involves the doping or co-doping of inorganic compounds mostly with lanthanide ions such as europium(III) [5] , [6] , [9] , [13] , [18] , [21] , [22] , whose scarcity [23] , [24] , [25] and supply disruption is a noticeable concern. From the materials science point of view, the main challenge is to develop a new ultraviolet downconverting metal activator-free phosphor that meets the requirements for WLEDs, namely high emission quantum yield, CRI>80 and thermal stability. Luminescent metal oxide nanoparticles may offer a possible alternative to meet the material demand for ultraviolet-pumped WLED, mainly because of their high stability, simplicity, low toxicity and low cost. The fluorescence properties of Al 2 O 3 or γ-AlOOH (boehmite) nanoparticles have already been studied [26] , [27] , [28] , [29] , [30] , [31] , [32] , [33] , [34] , [35] , [36] , [37] , [38] . For instance, these nanoparticles present emission in the ultraviolet and blue spectral regions due to lattice anion vacancies (F and F + centres or grouping of these two defects) [30] , [31] , [32] , [33] , [34] , [35] , [36] , [37] , [38] excited through absorption of anionic vacancies below 300 nm, mismatching the pumped wavelength (350–420 nm) of commercial ultraviolet chips [26] , [27] , [28] , [29] , [30] , [31] , [32] , [33] , [34] , [35] , [36] , [37] , [38] . Moreover, the typical emission quantum yield of Al 2 O 3 or γ-AlOOH nanoparticles is intrinsically very low, disabling any commercial application [36] . In this work, we report the possibility to sensitize the emission from boehmite point defects by a light harvesting chromophore leading to an enhancement of the emission quantum yield and to a lowering of the excitation energy. This is achieved by the development of hybrid organic–inorganic nanoparticles based on boehmite prepared by a one-pot non-aqueous approach. The synthesis relies on the ‘benzyl alcohol route’ [39] , [40] , [41] , [42] , [43] procedure involving the reaction of aluminium isopropoxide in benzyl alcohol at temperatures above 300 °C. The reaction procedure readily gives access to few-nm thick boehmite nanoplates capped with in situ -formed benzoate ligands. The advantage of these boehmite hybrid phosphors lies in the fact that they are made of non-toxic, abundant and low-cost materials that is desirable from an industrial and environmental viewpoint. Moreover, we demonstrate that a synergic energy transfer between the triplet levels of the organic phase and the F-centres of the inorganic component occurs. Thus, the as-formed hybrid nanoparticles exhibit high efficiency downconversion emission properties that cover most of the visible spectral region. By combining a near-ultraviolet chip and the boehmite hybrid nanoparticles, new transition metal- and lanthanide-free single-phase ultraviolet WLEDs have been fabricated. Characterization of γ-AlOOH hybrid nanoplates The structure of as-prepared samples has been determined by powder X-ray diffraction (XRD) ( Supplementary Fig. 1 ). The positions and the relative intensities of the XRD patterns match well with the boehmite crystal phase (JCPDS No. 21-1307 black line). The peaks located at 19.9° and 42.6° 2 θ (noted as star in some of the patterns) correspond to the formation of a low content of the hexagonal phase of aluminium oxide as secondary phase (JCPDS No. 04-007-2253). 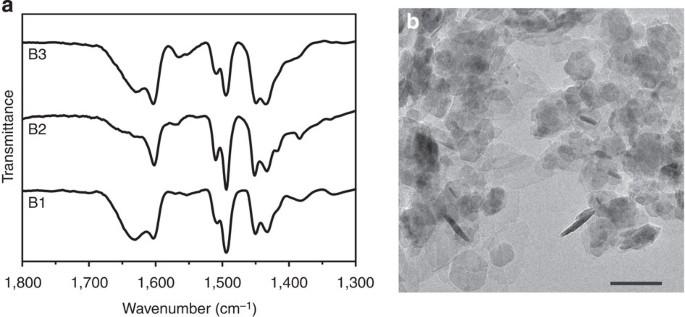Figure 1: FTIR and TEM characterization. (a) FTIR of the boehmite hybrid nanoparticles synthesized in benzyl alcohol at different reaction temperatures B1) 315 °C, B2) 325 °C and B3) 335 °C. (b) Representative TEM image of boehmite hybrid nanoparticles B1 (scale bar, 100 nm). The average crystallite sizes in the [010] and [001] directions, estimated from Rietveld refinement, increase with the reaction temperature (see Supplementary Table 1 and Supplementary Note 1 ). The boehmite structure was also confirmed by Fourier transform infrared spectroscopy (FTIR) ( Supplementary Fig. 2 and Supplementary Note 2 ). Vibrations of organic species absorbed onto boehmite nanoparticles are clearly visible in the 1,800–1,300 cm −1 range ( Fig. 1a ). The peaks at 1,602, 1,496 and 1,452 cm −1 appearing in all the samples are associated with the C=C stretching modes of the phenyl rings [41] , [42] , [43] . The two absorptions centred at 1,510 and 1,432 cm −1 are due to the asymmetric ( ν as ) and symmetric ( ν s ) stretching vibrations of carboxylate group (-COO − ) associated with the benzoate moieties bound to the particle surface. The energy difference between these two vibrations is 78 cm −1 pointing to the presence of a chelating bidentate coordination [44] , [45] . 13 C solid-state NMR is in good agreement with FTIR studies and indicates the presence of only benzoate species ( Supplementary Fig. 3 and Supplementary Note 3 ). The size and the morphology of the boehmite hybrid nanoparticles were characterized by transmission electron microscopy (TEM) ( Fig. 1b and Supplementary Fig. 4a–c ). They show platelet-like nanoparticles only few nanometres in thickness as determined from vertically aligned particles with respect to the electron beam. The platelet-like morphology is further confirmed by scanning electron microscopy (SEM) investigations ( Supplementary Fig. 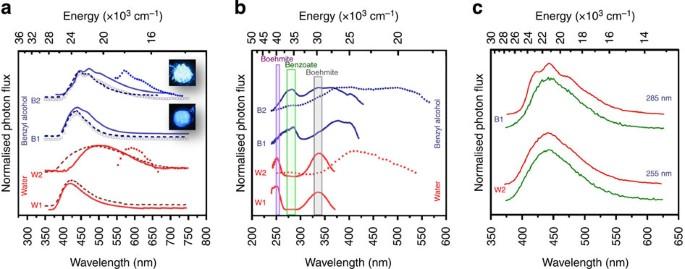Figure 2: Emission, excitation and time-resolved spectra. (a) Emission spectra (300 K) excited at 255 (dashed line), 285 (open circles), 360 (solid line) and 515 nm (solid circles) for boehmite hybrid nanoparticles synthesized in benzyl alcohol at 315 (B1) and 325 °C (B2) and boehmite nanoparticles synthesized in water (W1 and W2), inset ofa: photographs under ultraviolet excitation (365 nm) of B1 and B2. (b) Excitation spectra (300 K) monitored at 440 (solid line) and 600 nm (solid circles) for B1, B2, W1 and W2. (c) Time-resolved emission spectra (12 K) acquired at different SD values of 0.05 (red) and 50.0 ms (green) for B1 and W2 excited at 285 and 255 nm, respectively. 5a–c ) and Rietveld analysis of the XRD patterns ( Supplementary Table 2 and Supplementary Note 4 ). The latter shows that the average crystallite size along the [010] direction (so the stacking direction of the AlOOH layers) is considerably shorter than the in plane direction [001], which is the most typical signature of boehmite nanoplatelets as discussed in several articles [46] , [47] , [48] , [49] . Carbon, hydrogen and nitrogen (CHN) elemental analysis shows that the carbon content, and therefore the quantity of benzoate species attached to the particle surface generally increases with the reaction temperature ( Supplementary Table 1 and Supplementary Note 1 ). The oxidation of benzyl alcohol to benzoate species, which remain attached to the surface of the nanoparticles, controlling in some cases the particle growth and assembly behaviour, has been observed for rare earth sesquioxides, zirconium oxide and alkaline earth aluminate nanoparticles, when the reaction temperature exceeded ca. 250 °C (refs 40 , 41 , 42 , 43 ). In the present study, the role of benzoate species on the growth mechanisms of the hybrid nanoparticles is not as evident because boehmite nanoparticles of similar sizes could also be synthesized in water without the presence of benzoate ligands (Methods, Supplementary Figs 6–9 and Supplementary Note 5 ). These pure inorganic samples will be used as reference to assign the bands observed in the photoluminescence spectra of the hybrid nanoparticles. Figure 1: FTIR and TEM characterization. ( a ) FTIR of the boehmite hybrid nanoparticles synthesized in benzyl alcohol at different reaction temperatures B1) 315 °C, B2) 325 °C and B3) 335 °C. ( b ) Representative TEM image of boehmite hybrid nanoparticles B1 (scale bar, 100 nm). Full size image Optical properties Boehmite hybrid nanoparticles exhibit emission colour depending on the reaction temperature ( Fig. 2a ). Under ultraviolet excitation at 285 nm, the nanoparticles prepared at lower temperature (B1) display a broad emission band (full-width-at-half-maximum, FWHM, ca . 80 nm), in which three peaks at 417 (23,950 cm −1 ), 440 (22,725 cm −1 ) and 465 nm (21,500 cm −1 ) are superimposed on a large broad band ( Fig. 2a ). The energy difference between the peaks is ca. 1,225 cm −1 , which approximately corresponds to a resolvable vibrational fine structure originating from the triplet state of nπ * emissions of aromatic molecules [41] , [50] , [51] , [52] , [53] . At higher excitation wavelengths (355–405 nm), an increase in the relative intensity of the low-energy side of the emission spectra is detected ( Fig. 2a and Supplementary Fig. 10a ), readily suggesting that the boehmite phase is also contributing for the emission features (see below). By increasing the reaction temperature (B2 and B3), another component in the red region appears ( Fig. 2a and Supplementary Fig. 10b ), being ascribed, in the literature, to the presence of surface defects [26] , [27] , [35] , [37] . Figure 2: Emission, excitation and time-resolved spectra. ( a ) Emission spectra (300 K) excited at 255 (dashed line), 285 (open circles), 360 (solid line) and 515 nm (solid circles) for boehmite hybrid nanoparticles synthesized in benzyl alcohol at 315 (B1) and 325 °C (B2) and boehmite nanoparticles synthesized in water (W1 and W2), inset of a : photographs under ultraviolet excitation (365 nm) of B1 and B2. ( b ) Excitation spectra (300 K) monitored at 440 (solid line) and 600 nm (solid circles) for B1, B2, W1 and W2. ( c ) Time-resolved emission spectra (12 K) acquired at different SD values of 0.05 (red) and 50.0 ms (green) for B1 and W2 excited at 285 and 255 nm, respectively. Full size image For all the samples, the excitation spectra were monitored at 440 nm ( Fig. 2b and Supplementary Fig. 11 ), revealing the presence of four components in the ultraviolet at 255, 285, 340 and 365 nm. The excitation components at 285 and 365 nm have already been observed for analogous benzoate-capped nanoparticles [41] , [43] , being ascribed to the singlet excited states (S 2 and S 1 , respectively) of the phenyl rings. The components at 255 and 340 nm are assigned to the boehmite phase. Although in the solid state, absorption saturation effects may influence the intensity, the lower relative contribution of the boehmite-related components indicates that the main excitation path is through the benzoate-related states. The photoluminescence spectra of the model nanoparticles (W1, W2) confirm the interpretation of the spectra of the hybrid nanoparticles. The emission spectra of W1 is formed of a broad band (FWHM, ca . 80 nm) peaking at ca . 425 nm ( Fig. 2a and Supplementary Fig. 12a ), resembling that previously observed in boehmite [26] , [38] , Al 2 O 3 (refs 30 , 31 , 32 , 33 , 34 ) and Al-based [35] nanoparticles and assigned to lattice anionic oxygen vacancies (F or F + centres). When the crystallite size increases (W2), the emission spectrum becomes broader and shifts towards the red ( Fig. 2a and Supplementary Fig. 12b ), as observed for the hybrid nanoparticles (B2, B3 Fig. 2a and Supplementary Fig. 10b ). Comparing the excitation spectra of W1 with those of B1 ( Fig. 2b and Supplementary Fig. 13 ), two main conclusions can be drawn: (i) the components at 255 and 340 nm observed in the excitation spectra of the hybrid nanoparticles arise from the inorganic moiety and (ii) the absence of the 285 and 365 nm components (detected in the spectra of all benzoate-containing nanoparticles) further supports that such excitation components arise from the organic molecules. The emission quantum yield ( η yield ) was measured as a function of the excitation wavelength ( Supplementary Fig. 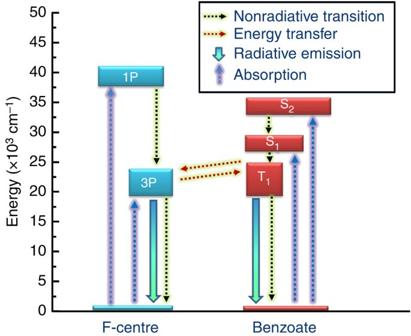Figure 3: Excitation and relaxation pathways diagram. Energy levels and possible relaxation pathways in the boehmite hybrid nanoparticles (B1). The energy position of the singlet (S1and S2) and triplet (T1) states relative to the benzoate were extracted from the previous analyses of the excitation spectrum and from the zero phonon line of the vibrational progression observed in the emission spectrum. The singlet (1P) and triplet (3P) energy values related to the F-centre correspond to the maximum intensity peak position of the components in the excitation and emission spectra of the W1 model nanoparticles, respectively. In all the cases, the width of the levels accounts for the FWHM of the bands in the emission and excitation spectra. 14 and Supplementary Table 3 ). The hybrid nanoparticles prepared at the lowest temperature (B1) show a maximum quantum yield value ( η yield =58±6%) that remains constant for excitation wavelengths between 280 and 380 nm. Because the quantum yield is independent of the excitation wavelength and the excitation at 280 nm is selective to the hybrid nanoparticles via the organic ligands, we conclude that the benzoate excited states play a major role in the enhancement of the emission quantum yield. Moreover, under excitation wavelengths related to the boehmite phase (such as, 260 nm and >400 nm) lower emission quantum yield values were measured ( Supplementary Fig. 14 and Supplementary Table 3 ). By increasing the reaction temperature, the maximum η yield decreases to 38±4% (B2) and 16±2% (B3). For the model compounds, lower η yield was measured for W1 (10±1%) and W2 (below 1%) ( Supplementary Fig. 14 and Supplementary Table 3 ). The decrease in the quantum yield as the nanoparticle size increases points to the appearance of competing non-radiative channels. Indeed, there are experimental evidences that when the nanoparticles size increases (both for the hybrid and inorganic ones), low-energy levels are created ( Fig. 2a ), which are competing non-radiative pathways. The substantially lower emission quantum yield of the model compounds highlights the role of the organic phase. In particular, due to the combination in a single material of organic light harvesting species (benzoate), the inorganic-related levels will be populated through the triplet sensitization mechanism [54] . The benzoate species act as antennas due to their high extinction coefficient in the ultraviolet spectral region (10 3 –10 4 M −1 cm −1 , Supplementary Fig. 15 ) extending the boehmite absorption range and increasing the absorption intensity ( Figs 2 and 3 ). After absorption by the high energy singlet state (S 2 ) of the benzoate species, S 2 →S 1 internal conversion occurs followed by S 1 →T 1 intersystem crossing that is favoured by the relative low-energy gap ( ca . 3,400 cm −1 ) between the S 1 and T 1 states. Due to the low energetic difference between the triplet state of the benzoate groups (T 1 ) and that of the boehmite (3P) (Δ E ≈450 cm −1 ), as well as a large spectral overlap between these states, an efficient energy transfer occurs ( Fig. 3 ). Figure 3: Excitation and relaxation pathways diagram. Energy levels and possible relaxation pathways in the boehmite hybrid nanoparticles (B1). The energy position of the singlet (S 1 and S 2 ) and triplet (T 1 ) states relative to the benzoate were extracted from the previous analyses of the excitation spectrum and from the zero phonon line of the vibrational progression observed in the emission spectrum. The singlet (1P) and triplet (3P) energy values related to the F-centre correspond to the maximum intensity peak position of the components in the excitation and emission spectra of the W1 model nanoparticles, respectively. In all the cases, the width of the levels accounts for the FWHM of the bands in the emission and excitation spectra. Full size image In addition to the near-resonance between the T 1 and 3P states, the high quantum yield is also due to an increase of the triplet radiative rate of the benzoate upon complexation with the nanoparticle surface. Density functional theory (DFT) calculations with inclusion of spin-orbit effects ( Supplementary Fig. 16 and Supplementary Note 6 ) indicate that the triplet radiative rate of the benzoate coordinated with Al atoms in a two tetrahedra model of the nanoparticle surface is ca . 13 times larger than the same rate in benzoic acid molecular crystals used to model the benzoate group coordinated with the Al atoms in the hybrid nanoparticles. 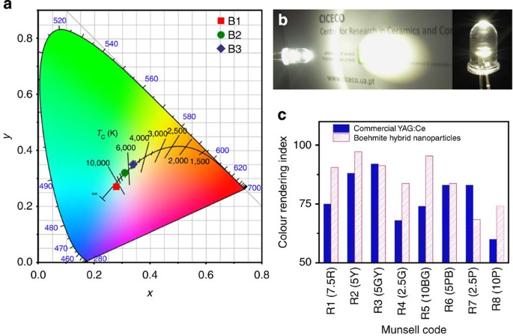Figure 4: Experimental results of the boehmite-based WLED device. (a) CIE chromaticity diagram (1,931) diagram showing the (x, y) emission colour coordinates of the boehmite hybrid nanoparticles excited at 390 nm (black dots are the colour points of illuminant D65 and illuminant A. The black solid curve is the Planckian locus, the CCT values are 9,882, 6,111, 4,811 and 4,849 K for B1, B2 and B3). (b) Photographs of the as-fabricated WLED with sample B2 operating at 3.0 V. (c) CRI of the B2-derived WLED and of a commercial YAG:Ce3+(390 nm) under forward-bias current of 20 mA. As a direct result of these two effects, the overall quantum yields of the boehmite hybrid nanoparticles B1 are the highest reported so far for ultraviolet-pumped white phosphors ( Supplementary Table 4 ), namely ZnSe:(Cu,Mn) quantum dots (13–17%) [2] , and higher than the figure of merit known for bulk organic–inorganic hybrid semiconductors (Zn 1.7 Cd 0.3 S 2 (hexylamine):Mn, 26–29%) [3] and white light-emitting Eu 3+ -doped Y 2 O 3 nanoparticles (19%) [21] . Benefiting from the above mentioned energy transfer mechanism, the quantum yield values reported here for the hybrid nanoparticles are much higher than for benzoate-capped ZrO 2 nanoparticles (<5%) [41] prepared by a similar route. In this system, although the energy of the benzoate is similar (22,500 cm −1 ), the energy levels of the ZrO 2 -related defects have a substantial higher energy (28,570 cm −1 ), disabling any efficient energy transfer process ( Supplementary Fig. 18 ). Time-resolved spectroscopy is a valuable tool to establish the presence of distinct emission components and to further study energy transfer processes. The use of cryogenics temperature (12 K) is fundamental to circumvent the contributions of thermally activated non-radiative pathways. The lifetimes associated with the various decay processes and the discussion of the different components are presented in Supplementary Information ( Supplementary Figs 19–24 ; Supplementary Table 5 and Supplementary Note 7 ). From these experiments, we can conclude that the emission features of the boehmite hybrid nanoparticles are mainly governed by the overlap of two distinct components arising from the triplet states of the benzoate species and F-centres. As illustrated in Fig. 2c , for the case of B1 nanoparticles, the 12 K emission spectrum acquired with a starting delay (SD) value of 0.05 ms is similar to those acquired in steady-state mode, exhibiting the vibrational progression fine structure (phenyl rings) and the F-centre components. For longer SD values (>2.00 ms), only the long-lived F-centre broad band emission is discerned ( Supplementary Fig. 19 ). This band is also detected in the emission spectra of W1 and W2 model nanoparticles ( Fig. 2c and Supplementary Fig. 19 ). The long-lived contribution (SD>2.00 ms) is characterized by an emission decay curve described by a bi-exponential function ( Supplementary Fig. 20 and Supplementary Table 5 ) ascribed to a first-order process followed by a second-order phosphorescence component typical of F-centres [6] , [7] , [8] , [9] , [10] , [11] , [12] . The lifetime value measured for the benzoate-related triplet states ( Supplementary Fig. 21 , τ =0.533±0.024 ms) is substantially lower than the typical long-lived emission (>1 ms) known for triplet states [41] , [42] , [43] . In particular, the triplet state lifetime value of benzoate molecules found for benzoate-capped ZrO 2 nanoparticles is also larger ( τ =9.2±0.8 ms) [41] . The decrease in the triplet lifetime is another argument in favour of the presence of energy transfer to the boehmite-related levels. The time-resolved emission spectra acquired at room temperature are similar to those measured at 12 K ( Supplementary Fig. 24 ), except for the decrease in the lifetime values of the benzoate triplet state to τ =0.237±0.001 ms ( Supplementary Fig. 21 ). A more detailed description of the mechanisms that assist such energy transfer processes was quantitatively discussed following the ideas proposed for the intramolecular energy transfer in coordination compounds. The calculation of the transfer rates mediated by exchange ( W ex ) and dipole–dipole ( W D–D ) mechanisms [55] ( Supplementary Table 6 ), yielded W ex =1.7 × 10 9 and W D–D =3.2 × 10 3 s −1 at a distance of 3 Å between the donor (benzoate triplet T 1 ) and acceptor (F-centre 3P) states. This distance may be considered the shortest one between the donor and acceptor. For larger separations, the dipole–dipole transfer rates are even less favourable ( Supplementary Note 8 ). This is a direct consequence of the high spectral overlap of the donor and acceptor triplet states. However, because the acceptors (F-centres) are defects in the nanoparticles, they would be at a wide range of distances from the donors (benzoates) and a distribution of energy transfer rates has to be considered. This results in an effective transfer rate ( W eff ) T 1 →3P that can be estimated from low temperature photoluminescence measurements. The back energy transfer rate 3P→T 1 ( W back ) is related to the forward rate ( W eff ) by the Boltzmann factor, that is, . At 12 K, it becomes insignificant, W back = e −647.5/ T W eff ≈10 −24 W eff , for an energy difference between the donor (T 1 ) and acceptor (3P) states of Δ E ≈450 cm −1 ( Fig. 3 and Supplementary Fig. 25 ). In addition, at 12 K, it may be assumed that the non-radiative decay rates from the 3P and the T 1 states are negligible. By solving the rate equations for the states shown in Fig. 3 ( Supplementary Figs 26–29 and Supplementary Note 9 ), the lifetimes of states 3P and T 1 can be obtained for a given set of transition rates. Using typical values for the absorption and intersystem transition rates, and assuming that W back =0 ( Supplementary Table 10 ), the calculated lifetimes ( Supplementary Figs 26 and 27 ) of states 3P (acceptor) and T 1 (donor) are 34 and 0.59 ms, respectively, when W eff =1,900 s −1 , k rad (3P)=25 s −1 and k rad (T 1 )=10 s −1 . These calculated values agree quite well with the experimental ones (40.00 and 0.53 ms). At room temperature, the back energy transfer rate is no longer negligible ( W back =0.12 × W eff ), which makes the states 3P and T 1 near resonant that significantly affects the emitting lifetime and populations [56] . Unfortunately, the calculated lifetime values at 300 K cannot be compared with the experimental ones because at this temperature ( Supplementary Figs 28 and 29 and Supplementary Note 10 ), non-radiative decaying rates are no longer negligible and care must be exercised when employing the usual relationships between lifetime and decaying rates [56] . Taken all together, spectroscopic data and calculations demonstrate the peculiarity of the boehmite hybrid nanoparticles because they combine an increase of the triplet radiative rate of the benzoate on complexation with Al at the surface of the nanoplates and the interplay between the populations of the triplet states at the benzoate and the boehmite F-centres (3P). The Commission International de l’Eclairage (CIE) colour coordinates, the CCT and the CRI values of the as-prepared boehmite hybrid nanoparticles are calculated as a function of the reaction temperature ( Fig. 4a , Supplementary Table 7 ). The hybrid nanoparticles (B2) exhibit CIE ( x , y ) coordinates of (0.32, 0.33) and a CCT of 6,111 K that match the properties of the CIE standard illuminant D65 (average daylight; CCT=6,500 K) [57] , with properties similar to that of cold white fluorescent bulbs with CCT values of ~6,000 K (refs 5 , 6 , 7 , 8 , 9 , 10 , 11 , 12 ). The hybrid nanoparticles prepared at higher temperatures (B3) show lower CCT values closer to the so-called ‘warm’ white light (CCT around 4,500 K) [5] , [6] , [7] , [8] , [9] , [10] , [11] , [12] . Figure 4: Experimental results of the boehmite-based WLED device. ( a ) CIE chromaticity diagram (1,931) diagram showing the ( x, y ) emission colour coordinates of the boehmite hybrid nanoparticles excited at 390 nm (black dots are the colour points of illuminant D65 and illuminant A. The black solid curve is the Planckian locus, the CCT values are 9,882, 6,111, 4,811 and 4,849 K for B1, B2 and B3). ( b ) Photographs of the as-fabricated WLED with sample B2 operating at 3.0 V. ( c ) CRI of the B2-derived WLED and of a commercial YAG:Ce 3+ (390 nm) under forward-bias current of 20 mA. Full size image The quantum yield of B2 hybrid nanoparticles was evaluated upon severe accelerated ageing tests performed under controlled relative humidity (RH) and temperature ( Supplementary Table 8 ). After 24 h, at 60 °C/RH=60% and at 25 °C/RH=95%, only minor changes in the quantum yield values were recorded. Under more severe testing conditions (RH=95% at 60 °C and RH=60% at 120 °C), a maximum decrease around 30–40% in the quantum yield value was observed. Nevertheless, after extra 72 h at 25 °C with RH=60%, the quantum yield values recover almost to the initial ones. Properties of the LED device The B2 hybrid nanoparticles were used to produce a WLED device by coating a commercial ultraviolet LED chip emitting at 390 nm ( Fig. 4b , Supplementary Fig. 30 ). The LED performance is typically characterized by the wall-plug efficiency (WPE, %), defined by the ratio between the radiant power (W) and the electrical power (W) and by the luminous efficacy (LE, lm/W), which accounts for the ratio between the luminous flux (lm) and the electric power (W). We should note, however, that a direct comparison of these values between distinct WLEDs must be taken with caution as they depend on the wall-plug efficiency of the ultraviolet-pumped LED and also on the device geometry. From the comparison between the performances of B2-based WLED and state-of-the-art lanthanide-based single phosphor ultraviolet WLEDs ( Supplementary Table 9 and Supplementary Note 11 ), the efficacy of the B2-derived WLED is among the best reported values. The radiant flux stability of the ultraviolet bare LED and B2-derived WLED was monitored for 1 week under continuous operation. After an initial decrease around 15% (ultraviolet LED) and of 35% (B2-derived WLED) in the first 40 h, it remains approximately constant ( Supplementary Fig. 31 ). CRI is the other important criteria for white light sources. Figure 4c compares the CRI values of the commercial-standard WLED using YAG:Ce 3+ as phosphor with those of B2-derived WLED. Our device shows a higher Ra (85.5) (average CRI value from R1–R8) due to the broad emission spectrum, compared with a Ra (79.0) of the commercial WLED. Moreover, the emission spectra (energy and FWHM) of our WLED are independent of the forward current (5–40 mA, Supplementary Fig. 32 and Supplementary Note 12 ) presenting, therefore, no colour shift under distinct working conditions, which is not the case for the YAG:Ce 3+ WLED [16] . Boehmite hybrid nanoparticles have been synthesized by a simple one-pot non-aqueous approach. They exhibit high efficiency and stable emission properties that can cover most of the visible region of the electromagnetic spectrum. The high quantum yield is due to an efficient and synergic energy transfer between the triplets states of the benzoate ligands and of the F-centres of the boehmite nanoplates. Through the combination of near-ultraviolet chips and these phosphorescent hybrid nanoparticles, transition metal and lanthanide-free ultraviolet WLEDs are fabricated. Finally, the findings reported here suggest that by modifying the organic and/or the inorganic components it would be possible to tune the optical properties of the hybrid nanoparticles by changing the absorption and emission properties of both counterparts while matching the respective energy levels. In particular, by employing alcohols with higher extinction coefficients and broader absorption spectra (such as 4-biphenyl methanol), blue LED chips may also be used. Another material design lesson learned from this study is that the thinner the boehmite nanoplates are, the higher the quantum yield is due to a minimization of non-radiative de-excitation pathways. Because the ‘benzyl alcohol route’ is particularly versatile with respect to the choice of the metal oxide that can be synthesized [40] and of the alcohol that can be employed for its synthesis [41] , [58] , [59] , the present work opens new perspectives for developing a large variety of photoactive metal oxide/carboxylate hybrid nanoparticles. Synthesis Boehmite hybrid nanoparticles: aluminium (III) isopropoxide (99.9%) and benzyl alcohol (99%) were purchased from Aldrich. All the reagents and solvents were used directly without further purification. The boehmite hybrid nanoparticles were synthesized following the benzyl alcohol route. The preparations were carried out in a glove box (O 2 and H 2 O <1 p.p.m. ), 500 mg of aluminium isopropoxide were added to 15 ml of benzyl alcohol in a glass vial. The glass vial was inserted into a steel autoclave and sealed carefully. The autoclave was removed from the glove box and heated in the oven at 315, 325 and 335 °C for 36 h (for B1, B2 and B3, respectively). The boehmite nanoparticles were synthesized using aluminium (III) isopropoxide and bidistilled water. All the preparations were carried out in air. For sample W1, 100 mg of aluminium isopropoxide were added to 5 ml of water in a pyrex vial. The vial was sealed with a Teflon cap and inserted in a CEM Discover SP microwave and processed at 175 °C for 10 min. For sample W2, 500 mg of aluminium isopropoxide were mixed with 25 ml of water in a glass vial and stirred for 15 min. The solution was transferred into a Teflon-lined steel autoclave and heated at 200 °C for 72 h. The resulting precipitates were centrifuged and washed thoroughly with ethanol and acetone. The powders were subsequently dried in air at 60 °C. Device design Fabrication of a prototype solid-state lighting device was prepared by removal of a LED lens from a commercial 390 nm excitation InGaAsN LED. Then, the lens surface was coated with a thin film by spin coating a cyanoacrylate solution of γ-AlOOH hybrid nanoparticles. The device was operated at 3.0 V. DFT calculations and rate equation simulations DFT calculations of the radiative rates for the triplet to singlet transitions were performed for benzoic acid (C 6 H 5 COOH) and benzoate coordinated with aluminium in a two tetrahedra (Tet2-benzoate) model of the nanoparticle surface. The equilibrium structures at the triplet state of these species were obtained with the B3LYP/6-31G(d) method. The starting geometries were distorted singlet planar benzoate structures and no symmetry constraints were imposed. The equilibrium structures are presented in Supplementary Fig. 16 . At the equilibrium triplet structure, the phosphorescence lifetimes were calculated with the self-consistent spin-orbit coupling (SOC) TDDFT (time-dependent DFT) method (SOC-TDDFT) including scalar relativistic effects through zero order regular approximation using the triple-zeta+polarization basis sets and the B3LYP functional [60] . The rate equations associated with the energy-level diagram in Fig. 3 were solved numerically by a fourth-order Runge–Kutta method with an adaptive integration step, where the initial populations of the ground states (F-centre and benzoate) were set to 1/2 and zero for the other states [61] . These equations were propagated up to 0.1 s and the steady-state populations were used as the starting populations for a new propagation to determine the lifetimes [56] . Characterization techniques Powder XRD was performed in the Bragg–Brentano geometry using a PANalytical X’Pert and PANalytical Empyrean powder diffractometers equipped with Cu Kα radiation (154.18 pm) and set to 45 kV/40 mA. Both machines were calibrated using NIST LaB 6 powder. Data for the Rietveld refinement were collected in the range 5<2 θ <70° with a step of 0.2°. For TEM measurements, one or two drops of the solution of the nanoparticles in ethanol were deposited on a copper grid coated with an amorphous carbon film. A Philips CM200 microscope operated at 200 kV was used. SEM investigations were carried out using a high-resolution SEM Hitachi SU-70 operated between 2 and 30 kV acceleration voltage. FTIR measurements were carried out on a Bruker Optics Tensor 27 spectrometer in the range 4,000–350 cm −1 in transmission mode. The pellets were prepared by adding 1–2 mg of nanoparticles powder to 100 mg of KBr. The mixture was carefully homogenized and compressed with a uniaxial pressure of 9 MPa. CHN elemental analyses were performed using a CHNS-932 elemental analyser with standard combustion conditions and handling of the samples in air. The organic ligands attached to the surface of the particles on drying were also analysed by solid-state NMR on a BRUKER AVANCE 400 spectrometer equipped with a 2.5 mm CP/MAS probe. Optical studies The photoluminescence spectra were recorded at room temperature and at 12 K with a modular double grating excitation spectrofluorimeter with a TRIAX 320 emission monochromator (Fluorolog-3, Horiba Scientific) coupled with a R928 Hamamatsu photomultiplier, using a front face acquisition mode. The excitation source was a 450 W Xe arc lamp. The emission spectra were corrected for detection and optical spectral response of the spectrofluorimeter and the excitation spectra were corrected for the spectral distribution of the lamp intensity using a photodiode reference detector. The time-resolved spectroscopy (emission spectra and emission decay curves) was measured at 12 K and room temperature with the setup described for the luminescence spectra using a pulsed Xe–Hg lamp (6 μs pulse at half width and 20–30 μs tail). At room temperature, time-resolved spectroscopy was also recorded on a Fluorolog TCSPC spectrofluorimeter (Horiba Scientific) coupled with a TBX-04 photomultiplier tube module (950 V), 200 ns time-to-amplitude converter and 70 ns delay. The excitation source was a Horiba–Jobin–Yvon-pulsed diode emitting at 390 nm (NanoLED-390, 1.2 ns pulse duration, 1 MHz repetition rate and 150 ns synchronization delay), Supplementary Fig. 24b . The absolute emission quantum yield values were measured at room temperature using a quantum yield measurement system C9920-02 from Hamamatsu. This system consists of a Xe arc lamp (150 W), a monochromator (bandwidth 2 nm, an integrating sphere made of Spectralon) (99% reflectance for wavelengths within 350–1,650 nm) with inner diameter of 84 mm and a multichannel detector (wavelength resolution <2 nm). The emission quantum yield ( ϕ ) is given by where N Abs and N Em are the number of photons absorbed and emitted by a sample, respectively, h is Planck’s constant, c is the velocity of light, and are the emission intensities of the measured with and without a sample, respectively, in the emission spectra wavelength interval ( λ 1 , λ 2 ) and and are the integrated intensities of the excitation radiation measured with and without a sample, respectively, in the excitation wavelength interval ( λ 3 , λ 4 ). To validate the calculation methodology, the emission quantum yield of a 1 mm thick pellet of the white standard sodium salicylate (Merck P.A.) and of the commercial YAG:Ce 3+ (YAG 432, Hung TA Trading Co. Ltd) was also measured under the same experimental conditions. The emission quantum yield value measured for sodium salicylate was 56% excited at 360 nm and those measured for YAG:Ce 3+ were 95% excited at 340 and 460 nm. The reproducibility of the measurement was tested by performing three measurements for each sample revealing s.d. below 0.5%. The measurement accuracy is within 10% according to the manufacturer. Photostability tests The emission spectra, the CIE colour coordinates and the emission quantum yield were evaluated after the hybrid samples being placed inside a climatic chamber (Angelantoni Industrie, model Challenge 340). The hybrid nanoparticles were subjected at distinct test conditions at constant temperature ( T ) and RH values, namely, T =25 °C/RH=95%; T =25 °C/RH=95%; T =120 °C/RH=60% and T =25 °C/RH=95%. The accuracy is 0.3 °C and 3%. Each test has the duration of 24 h. The emission spectra were measured with the spectrofluorimeter and integrating sphere above mentioned for the measurement of the photoluminescence and quantum yield, respectively. The WLED device performance was evaluated over ca . 200 h under continuous operation at 3 V. The radiant flux (W) and the luminous flux (lm) of the WLED and of the bare ultraviolet LED were measured using an integrating sphere ISP 150L-131 from Instrument Systems. The integrating sphere (BaSO 4 coating) has internal diameter of 150 mm and was coupled to an array spectrometer MAS 40 from Instrument Systems. The measurements are accurate within 5%, accordingly to the manufacturer. How to cite this article : Bai, X. et al. Efficient and tuneable photoluminescent boehmite hybrid nanoplates lacking metal activator centres for single-phase white LEDs. Nat. Commun. 5:5702 doi: 10.1038/ncomms6702 (2014).